A combined experimental and theoretical study on the reactivity of nitrenes and nitrene radical anions Nitrene transfer reactions represent one of the key reactions to rapidly construct new carbon-nitrogen bonds and typically require transition metal catalysts to control the reactivity of the pivotal nitrene intermediate. Herein, we report on the application of iminoiodinanes in amination reactions under visible light photochemical conditions. While a triplet nitrene can be accessed under catalyst-free conditions, the use of a suitable photosensitizer allows the access of a nitrene radical anion. Computational and mechanistic studies rationalize the access and reactivity of triplet nitrene and nitrene radical anion and allow the direct comparison of both amination reagents. We conclude with applications of both reagents in organic synthesis and showcase their reactivity in the reaction with olefins, which underline their markedly distinct reactivity. Both reagents can be accessed under mild reaction conditions at room temperature without the necessity to exclude moisture or air, which renders these metal-free, photochemical amination reactions highly practical. Photochemistry is a classic discipline in chemistry and early reports date back even to the beginning of the 20 th century forecasting the potential of photochemical synthesis on the challenges of modern societies [1] . It features light as the main source of energy to conduct chemical transformations and can thus be regarded as a key pillar in the development of sustainable approaches and reduced ecological footprint. Today, photochemistry is one of the most rapidly developing fields in chemistry and the past decades witnessed the development of major milestones and concepts, such as dye-sensitized solar cells [2] , polymerization chemistry [3] , protein labeling [4] , photoredox catalysis [5] , [6] , [7] , [8] , and classic photochemical applications [9] , [10] , [11] that leverage photochemistry as one of the key technologies in the advancement of all chemical disciplines. In organic synthesis, photochemistry constitutes an important strategy to access reactive intermediates via excited state chemistry of catalysts [5] , [6] , [7] , [8] or reagents [11] , [12] , [13] , [14] . Significant advances have been made in the context of organic synthesis methodology, for example in the utilization of radicals in the presence of photoredox catalysts [5] , [6] , [7] , [8] or carbenes via the photolysis reaction of appropriate reagents [11] , [12] , [13] , [14] . The access and application of nitrenes [15] , [16] , [17] , [18] , [19] , [20] , [21] , [22] or analogs therof [23] under visible light photochemical conditions however remains largely underestimated although it would allow for direct amination reactions with vast potential in modern drug synthesis [21] , [22] . Such photochemical nitrene transfer reactions would significantly expand currently available concepts in classic metal-catalyzed nitrene transfer reactions (Fig. 1a ) and provide pathways under mild conditions to the pivotal nitrene intermediate. Today, essentially two strategies have been developed to access nitrenes under photochemical conditions. One concept harnesses the use of metal-catalyzed nitrene transfer reactions under UV light photochemical conditions to facilitate the formation of metal-nitrene intermediates (Fig. 1b ) [24] , [25] , [26] , [27] , [28] . Another concept employs highly specialized, tailor-made nitrene transfer reagents ( 7 ), relying on strong UV-light for their photolysis [29] . UV-light can however significantly reduce reaction efficiency and increase by-product formation. Yet, UV light still remains a prerequisite to access pivotal (metal-)nitrene intermediate under photochemical conditions (Fig. 1b ). The use of visible light is thus in high demand to overcome these limitations, to enable sustainable nitrene transfer reactions and to develop strategies for amination reactions (Fig. 2 ). Fig. 1: Photochemical amination reactions with nitrenes. a Classic precursors of nitrenes. b Previous applications of UV light-mediated or assisted nitrene transfer reactions. Full size image Fig. 2: Photochemical amination reactions with nitrenes. a Photochemical properties of iminoiodinane 1a and computed HOMO and LUMO. b Comparative study of nitrene vs. nitrene radical anions. c Key features of this work. Full size image In this context, our group recently reported an initial application of nitrene radical anions in organic synthesis [30] . Their initial discovery dates back to 1980, when MacDonald described the synthesis of the phenyl nitrene radical anion [23] . Applications in organic synthesis however remained scarce and detailed, comparative studies on the properties of nitrene and nitrene radical anion remain elusive. Such studies would allow for fundamental understanding of similarities and differences of chemical properties and reactivity of these monovalent, nitrogen-based reactive intermediates and can provide the basis for further development of metal-free amination reactions (Fig. 2 ). In this work, we show that iminoiodinanes are suitable, bench-stable reagents that can be used to access either a triplet nitrene or a nitrene radical anion intermediate under photochemical or photocatalytic conditions, respectively. We showcase the reactivity of these monovalent nitrogen-based reactive intermediates in the reaction with olefins that can lead either to aziridination or C-H amination reactions. Experimental and computational studies are discussed to rationalize for the observed experimental data. Reaction optimization The utilization of simple, readily available nitrene transfer reagents can be regarded as a prerequisite for the realization of photochemical amination reactions. We therefore decided to initially study the photochemical properties of iodinane 1 and phenyl azide, which are commonly applied reagents in metal-catalyzed nitrene transfer reactions. While phenyl azide did not show absorbance in the visible light region, a range of different, readily available iminoiodinanes 1 revealed a weak absorbance in the visible light region as determined by both experiment and theory (Fig. 2a and Supplementary Fig. 1 ). An important observation was made for the electron distribution of the HOMO and LUMO. While the HOMO of 1a is predominantly associated to electron density at the nitrogen atom (Fig. 2a ), the electron distribution in the LUMO is shifted to the iodine atom (Fig. 2a and Supplementary Fig. 6 ), which could facilitate photolysis reactions and formation of nitrene intermediates. 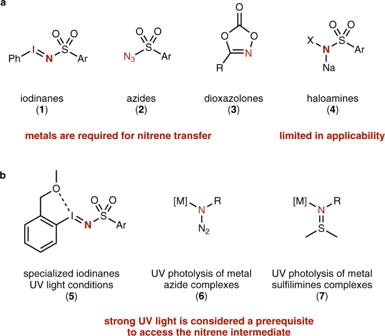Fig. 1: Photochemical amination reactions with nitrenes. aClassic precursors of nitrenes.bPrevious applications of UV light-mediated or assisted nitrene transfer reactions. Based on this observation, we investigated the reaction of α-methyl styrene 12a with iminoiodinane 1a under photochemical conditions (Table 1 ). Indeed, a very efficient amination reaction was observed in the presence of blue light (470 nm) that lead to the selective formation of the C-H functionalization product 10a without accompanying by-products from aziridination ( 11a ). Other light sources proved by far less efficient, which might be related to weaker absorption or side-reactions due to the high-energy UV light. A surprising observation was made when switching to photocatalytic reaction conditions. Using simple [Ru(bpy) 3 ]Cl 2 as photocatalyst, a complete reversal of reactivity was observed and selective aziridination reaction to yield 11a occurred. Other photocatalysts, such as [Ru(bpz) 3 ](PF 6 ) 2 , iridium-based photocatalysts, or organic dyes did not alter the reactivity and the C-H functionalization product 10a was formed selectively. Only in the case of Eosin Y as photocatalyst, a mixture of C-H amination ( 10a ) and aziridination ( 11a ) was observed. Further optimization steps included investigations on the solvent, concentration, reaction stoichiometry, yet no further improvements were observed (Supplementary Table 1 ). Table 1 Investigations on the photochemical and photocatalytic reaction iminoiodinane 1a with α-methyl styrene 12a . Full size table Comparative study on the reaction mechanism To further explore this divergent reactivity, we examined control experiments to provide an understanding of the underlying reaction mechanism. No notable association of α-methyl styrene 12a or phenyl iodide with iminoiodinane 1a were observed by 1 H-NMR studies, suggesting no association of reagents. Similarly, no notable decomposition of phenyl iodide under 470 nm blue light irradiation was observed within 4 h, which suggests that iodine species do not participate as hidden catalysts in the reaction. Further studies on the reaction mechanism involved theoretical calculations to better rationalize this photochemical nitrene transfer reaction (Fig. 3 ). We therefore conducted calculations using (TD)-DFT methods to rationalize the photochemical reaction of iminoiodinane 1a and DFT methods for the catalytic reaction involving photosensitizers. These calculations reveal that photochemical excitation of 1a leads to formation of an excited state 1a* that remains in singlet state. This excited state can now undergo two different pathways: A) relaxation on the singlet spin surface leads to the direct formation of a singlet nitrene that features a very short N-O distance, which can be interpreted as a stabilization of the low-valent nitrene with the lone pair of an oxygen atom of the pendant sulfonyl group. B) relaxation involving intersystem crossing (ISC) results in the formation of a triplet intermediate 1a-T , which features a very long N-I bond, close to a non-bonding situation. Scanning of different N-I bond lengths indicated that further elongation of the N-I bond proceeds in a barrier-free fashion to directly lead to a triplet nitrene intermediate. This triplet nitrene intermediate is the energetically favored intermediate and can alternatively be accessed from the high-lying singlet nitrene via intersystem crossing. This theoretical analysis of the photochemistry of iminioiodinane 1a now rationalizes for the formation of a triplet nitrene intermediate under photochemical conditions and shows a marked difference to the ground state reactivity [31] . Under photocatalytic conditions, calculations are in line with our previous report [30] and a very facile reduction of the iodinane, leading to iodinane radical anion INT1 . This anion features a very long N-I bond that is close to non-existent and therefore a rapid cleavage of the N-I bond can occur in a barrierless process to give a nitrene radical anion. Fig. 3: theoretical calculations on the formation of the nitrene intermediate; calculations were performed at the SMD(DCM)-(U)M06-2X-D3/def2-TZVP//(U)M06-2X-D3/def2-SVP level of theory. Gibbs energies are given in kcal mol −1 . Full size image For further analysis and understanding of the reactivity of triplet nitrene and nitrene radical anion, we examined their structural and electronic properties. The calculations show that the nitrene radical anion possesses a higher electron density at the nitrogen atom compared to the triplet nitrene, which in turn leads to higher nucleophilicty of the nitrene radical anion (Supplementary Figs. 4 , 7 , and 8 ). For stabilization of the negative charge, the sulfonyl group plays an important role as an electron acceptor leading to mesomeric stabilization of the nitrene radical anion. The aromatic ring plays only a minor role in stabilization of the nitrene radical anion. The analysis of bond lengths further supports this mesomeric effect within the nitrene radical anion. Despite of the additional negative charge, the S-N bond shortens upon formal reduction from triplet nitrene to nitrene radical anion from 1.71 Å to 1.56 Å and thus resembles more an S-N double bond in the case of the nitrene radical anion, which is also reflected by bond order analysis (Supplementary Fig. 5 ). Further exploration concerned the evaluation of the reaction mechanism and an understanding of the distinct reactivity of triplet nitrene and nitrene radical anion by theory and experiment (Fig. 4 ). In the case of the triplet nitrene, we examined two different reaction pathways using DFT calculcations (Fig. 4a , right). A first pathway involves hydrogen atom transfer from α-methyl styrene to the triplet nitrene intermediate, yet an activation free energy of 14.7 kcal mol −1 and the formation of two separate radicals that need intermolecular radical recombination renders this pathway not feasible (Supplementary Fig. 11 , TS6 ). A second pathway involves the addition of the triplet nitrene to α-methyl styrene via a TS3 with an activation free energy of only 6.1 kcal mol −1 , which is significantly favored over the hydrogen transfer pathway. This addition product can undergo intersystem crossing to give an open shell singlet species that can either cyclize to give the aziridine 11a , or undergo hydrogen atom transfer to give the C-H functionalization product 10a . Analysis of the respective transition states reveals significant steric hindrance of rotation around the central C-C bond, which renders cyclization energetically unfavorable over hydrogen atom transfer. The latter is favored by 2.5 kcal mol −1 and now reasons the reactivity of triplet nitrene intermediates with α-methyl styrene to yield the C-H functionalization product 10a . Further studies concerned the reaction of the nitrene radical anion (Fig. 4a , left). In this case, the radical addition to the olefin occurs with a significantly higher activation free energy as compared to the triplet nitrene, which is reasoned by higher electron density. Subsequent reduction by the oxidized state of the photoredox catalyst furnishes a zwitterionic intermediate INT4 that quickly undergoes cyclization to give the aziridine product 11a (Supplementary Fig. 10 ). Fig. 4: Control experiments and theoretical calculations on the formation of the nitrene intermediate; calculations were performed at the SMD(DCM)-(U)M06-2X-D3/def2-TZVP//(U)M06-2X-D3/def2-SVP level of theory. a Energy surface of the reaction of triplet nitrene and nitrene radical anion. Gibbs energies are given in kcal mol −1 . b Reaction with deuterated α-methyl styrene. c Reaction with α-ethyl styrene. d Photocatalytic reaction with β-methyl styrene. 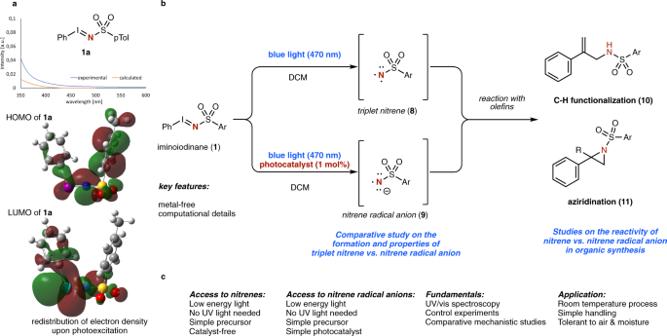Fig. 2: Photochemical amination reactions with nitrenes. aPhotochemical properties of iminoiodinane1aand computed HOMO and LUMO.bComparative study of nitrene vs. nitrene radical anions.cKey features of this work. e Photochemical reaction with β-methyl styrene. 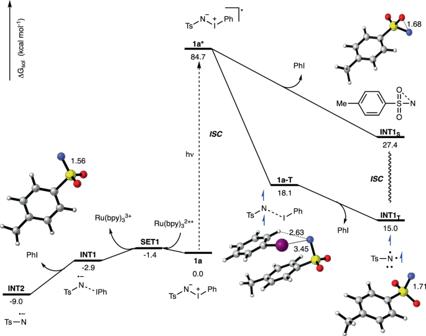Fig. 3: theoretical calculations on the formation of the nitrene intermediate; calculations were performed at the SMD(DCM)-(U)M06-2X-D3/def2-TZVP//(U)M06-2X-D3/def2-SVP level of theory. Gibbs energies are given in kcal mol−1. Full size image To examine the above pathways experimentally, we first probed the reaction mechanism with α-trideuteriomethyl styrene 12a- d 3 under the optimized reaction conditions (Fig. 4b ). The deuterium content was fully preserved under both photochemical and photocatalytic conditions. Furthermore the aziridine was selectively formed and the trideuteriomethyl-substituted aziridine 11a- d 3 was obtained as the sole reaction product. In the case of the photochemical reaction, the deuterium label was found exclusively in the olefinic position of the reaction product, thus supporting the addition mechanism. Studies on the reaction kinetics of 12a and 12a- d 3 revealed only a very small kinetic isotope effect, which suggests that the hydrogen atom transfer does not occur in the rate determining step, as suggested by the theoretical calculations (Fig. 4b , and Supplementary Fig. 3 ). Further control experiments involved the reaction of α-ethyl styrene (Fig. 4c ). While selective aziridination was observed under photocatalytic reaction conditions, a mixture of different products ( 15 – 18 ) that can arise from an addition – hydrogen atom transfer mechanism were observed under photochemical conditions. The theoretical analysis of reaction pathways for the hydrogen atom transfer revealed that pathways involving different hydrogen atom transfer can occur due to the presence of the ethyl group. These are very similar in energy and thus reason the unselective reaction and represent a limitation of the present C-H amination method in the case different hydrogen atom transfer reactions are possible (Supplementary Fig. 14 ). When studying both individual isomers of β-methyl styrene ( Z -19 and E -19 ), we could observe a selective reaction towards the trans -aziridine 20 , which is indicative of a stepwise mechanism under both photochemical and photocatalytic reaction conditions. Further control experiments involved the use of spin trapping reagents, such as 2,2,6,6-Tetramethylpiperidinyloxyl (TEMPO), 5,5-dimethyl-1-pyrroline-1-oxide (DMPO), or DNP, and in all cases a complete suppression of the photochemical and photocatalytic reactions were observed, which is indicative of radical intermediates or participating in the reaction mechanism (Supplementary Tables 2 and 3 ). Application in synthesis We next turned our attention towards applications of the above protocols in amination reactions (Fig. 5 ). The photochemical C-H functionalization reaction of α-methyl styrenes 12 proceeded smoothly and the allylamine products 10a–q were obtained in good isolated yield, without formation of by-products from aziridination (Fig. 5a ). Halogens, electron-withdrawing or -donating groups in all positions of the aromatic ring were compatible and the corresponding products were obtained in high isolated yields ( 10a – o ). Importantly, ortho -substitution ( 10 m, n ) had a slightly detrimental effect on the product yield. Similarly, different sulfonyl groups were tolerated under the present photochemical reaction conditions and the allyl amines products were obtained in high isolated yield ( 10p, q ). When applying this photochemical protocol to cyclic, trisubstitued, cyclic olefins, 1-alkynyl-1-methyl or aliphatic 1,2-disubstituted olefins, the C-H amination products 10r – v were selectively obtained in good isolated yield. Then, the photocatalytic protocol was employed in the aziridination of α-methyl styrenes (Fig. 5b ). We examined a similar range of substituents, including halogen, alkyl, cyano, ether or alkoxy substituents, at both the sulfonyl group and the benzene ring of the α-methyl styrene, which proved compatible under photocatalytic conditions. Only in the case of ortho -substitution slightly reduced reaction yields were obtained ( 11i – k ). Most notably, in this case also different α-alkyl-substituted styrene derivatives, such as a very bulky tert .-butyl group ( 11s ), and nucleophilic N -heterocycles ( 11p , q ) were well tolerated to yield the corresponding aziridines in high yield, which are commonly very challenging substrates in aziridination reactions. Furthermore, a range of trisubstitued, cyclic olefins, and further examples of 1,1-disusbtituted olefins were studied under the present photocatalytic conditions to yield the aziridine products 11t – 11ad . Fig. 5: Scope of the nitrene transfer reactions in the photochemical C-H functionalization and photocatalytic aziridination reaction via nitrene radical anions. a Photochemical reaction with α-methyl styrenes. 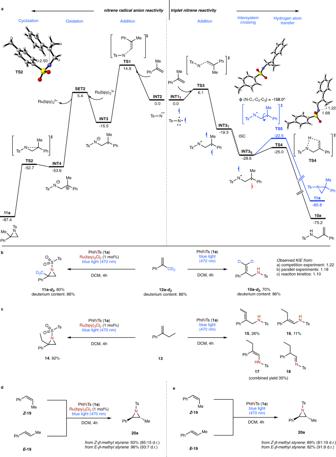Fig. 4: Control experiments and theoretical calculations on the formation of the nitrene intermediate; calculations were performed at the SMD(DCM)-(U)M06-2X-D3/def2-TZVP//(U)M06-2X-D3/def2-SVP level of theory. aEnergy surface of the reaction of triplet nitrene and nitrene radical anion. Gibbs energies are given in kcal mol−1.bReaction with deuterated α-methyl styrene.cReaction with α-ethyl styrene.dPhotocatalytic reaction with β-methyl styrene.ePhotochemical reaction with β-methyl styrene. b Photocatalytic reaction with α-methyl styrenes. Full size image Finally, we embarked on the reaction of simple styrene derivatives under both photochemical and photocatalytic conditions (Fig. 6 ). In both cases, aziridination reaction was observed in high yields, with the photocatalytic reaction being slightly superior over the photochemical reaction. Different sulfonyl groups as well as a range of electronically and sterically distinct substituents at the aromatic ring of the styrene component proved compatible ( 22a – t ). Most notably, even in the presence of two sterically demanding ortho -chloro substituents ( 22t ) the desired aziridine product was obtained in good isolated yield. Further studies involved the reaction of cyclic olefins, such as indene, which smoothly reacted to the aziridine product ( 22 u ) in high isolated yield. An important difference in the reactivity of nitrene and nitrene radical anion was however observed in the reaction with aliphatic olefins (Fig. 6b ). While only a poor yield was obtained under photochemical conditions, the photocatalysis approach via the nitrene radical anion proved superior and high yield in the aziridination reaction of aliphatic olefins was observed ( 23a – i ). Further examples under investigation concerned the utilization of 1,2-disubstituted olefins. In this case, different aryl-alkyl and alkyl-alkyl disubstituted olefins smoothly underwent selective aziridination reaction to afford the trans -azridines 20a–i in high yield. Fig. 6: Scope of the photochemical and photocatalytic nitrene transfer reactions with styrenes and aliphatic olefins. a Evaluation of styrene derivatives. b Evaluation of aliphatic olefins c evaluation of 1,2-disubstituted olefins. Full size image The aziridination was then examined by DFT calculations, which suggest a similar pathways as in the aziridination reaction of α-methyl styrene for both photochemical and -catalytic conditions (cf. Fig. 3 and Supplementary Figs. 12 , 13 ). However, a distinct difference in the conformational flexibility of the diradical intermediate INT3 S (cf. Fig. 4a , right) was observed. The absence of the α-methyl group renders the cyclization step to the aziridine much more favorable and it can proceed with a very low activation free energy of only 1.4 kcal mol −1 . The direct comparison of the respective transition states show that the α-methyl group results in a conformational twist and that prevents efficient aziridination as it can be seen in the torsional angle around the N-C-C-C Ar bond (Supplementary Fig. 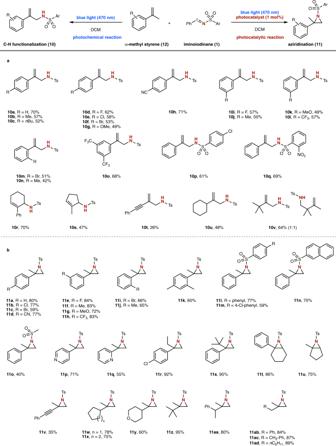Fig. 5: Scope of the nitrene transfer reactions in the photochemical C-H functionalization and photocatalytic aziridination reaction via nitrene radical anions. aPhotochemical reaction with α-methyl styrenes.bPhotocatalytic reaction with α-methyl styrenes. 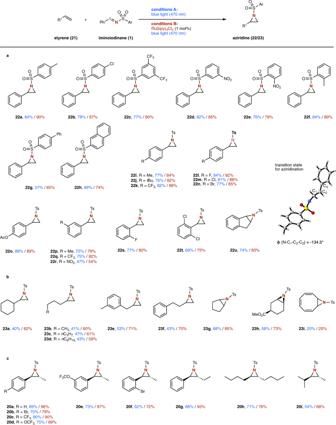Fig. 6: Scope of the photochemical and photocatalytic nitrene transfer reactions with styrenes and aliphatic olefins. aEvaluation of styrene derivatives.bEvaluation of aliphatic olefinscevaluation of 1,2-disubstituted olefins. 11 ). In summary, we herein report on amination reactions of olefins with iminoiodinane reagents under purely photochemical and photocatalytic reaction conditions. Depending on the reaction conditions, these amination reactions proceed via chemically distinct monovalent, nitrogen-based reactive intermediates that in turn lead to different reaction products in the reaction with α-methyl styrenes. While triplet nitrenes can be accessed via direct photolysis of iminioiodinanes and lead to C-H functionalization, a nitrene radical anion is formed under photocatalytic conditions and leads to aziridination reaction. We studied the formation, properties, and reactivity of triplet nitrene and nitrene radical anion using computational calculations to rationalize the observed reactivity in the reaction with olefins, which was further validated in control experiments. We conclude with studies on the application of these amination reactions in the reaction with a diverse set of olefins, ranging from α-substituted styrenes, styrenes, towards aliphatic olefins. General method for the photochemical reactions In an oven-dried tube (10 mL), equipped with a magnetic stirring bar, iminoiodinane (0.2 mmol, 1.0 equiv) and alkene (5.0 equiv) are dissolved in 2 mL DCM under air atmosphere. The reaction is stirred and irradiated with a 3 W LED lamp (5 cm distance) for 4 h. A cooling fan is used to maintain room temperature (25–28 °C). The product was obtained after column chromatography using n -hexane/EtOAc as eluent. General method for the photocatalytic reactions In an oven-dried tube (10 mL), equipped with a magnetic stirring bar, iminoiodinane (0.2 mmol, 1.0 equiv), alkene (5.0 equiv), and catalyst (1 mol%) are dissolved in 2 mL DCM under air atmosphere. The reaction is stirred and irradiated with a 3 W LED lamp (5 cm distance) for 4 h. A cooling fan is used to maintain room temperature (25–28 °C). The product was obtained after column chromatography using n -hexane/EtOAc as eluent. Computational details All calculations were performed using the Gaussian 16 series of programs [32] . All structures were optimized at the (U)M06-2X level [33] of theory in combination with D3 dispersion corrections [34] , in which all atoms were described with the def2-SVP basis set [35] . Analytical frequency calculations were carried out at the same level of theory in order to confirm each stationary point as either an intermediate (no imaginary frequencies) or a transition state (only one imaginary frequency). Key transition-state structures were confirmed to connect corresponding reactants and products by intrinsic reaction coordinate (IRC) calculations [36] , [37] . The electronic energy was then refined using def2-TZVP basis set [35] at the (U)M06-2X level on the optimized geometries in combination with D3 dispersion corrections. Solvation energies in dichloromethane (ε = 8.93; for acetonitrile: ε = 35.688) were evaluated by IEFPCM calculations with radii and non-electrostatic terms for SMD solvation model [38] based on the optimized structures. Time-dependent (TD)-DFT calculations were carried out on the optimized structures of the PhINTs to obtain the absorption wavelength.